Regulation of MITF stability by the USP13 deubiquitinase The microphthalmia-associated transcription factor (MITF) is essential for melanocyte development. Mutation-induced MAPK pathway activation is common in melanoma and induces MITF phosphorylation, ubiquitination, and proteolysis. Little is known about the enzymes involved in MITF ubiquitination/deubiquitination. Here we report the identification of a deubiquitinating enzyme, named ubiquitin-specific protease 13 (USP13) that appears to be responsible for MITF deubiquitination, utilizing a short hairpin RNA library against known deubiquitinating enzymes. Through deubiquitination, USP13 stabilizes and upregulates MITF protein levels. Conversely, suppression of USP13 (through knockdown) leads to dramatic loss of MITF protein, but not messenger RNA. Through its effects on MITF deubiquitination, USP13 was observed to modulate expression of MITF downstream target genes and, thereby, to be essential for melanoma growth in soft agar and in nude mice. These observations suggest that as a potentially drugable protease, USP13 might be a viable therapeutic target for melanoma. The microphthalmia-associated transcription factor (MITF) is a member of the basic helix-loop-helix-leucine zipper transcription factor family and is a key regulator of development and survival for melanocytes as well as melanoma [1] . The protein encoded by the MITF gene activates the transcription of numerous pigment cell-specific genes [2] . Recent reports suggest that amplification of MITF is oncogenic in 10–20% of melanomas [3] . Additionally, inhibition of MITF appears to cause melanoma cell death regardless of its amplification, presumably due to its lineage survival requirement [2] , [4] , [5] . Because of MITF's role as a melanoma oncogene, or its lineage-specific role as a master regulator of melanocyte development, its activity appears to be required for survival of nearly all melanomas studied to date. The activity and expression of MITF are regulated by a variety of mechanisms including transcriptional regulation, targeting by micro RNA, and post-translational modifications. For example, α-melanocyte-stimulating hormone strongly increases MITF expression through a cyclic AMP and CREB/ATF1-mediated pathway [6] , [7] , [8] . In addition, through its melanocyte-specific promoter (M-MITF), the expression of MITF is regulated by paired box gene 3 (PAX3), SRY (sex-determining region Y)-box 10 (SOX10), lymphoid enhancer-binding factor 1 (LEF1), and one cut domain 2 (ONECUT-2) [9] , [10] , [11] , [12] In Clear Cell Sarcoma the EWS-ATF1 fusion oncoprotein occupies the MITF promoter, constitutively replaces the cAMP-driven activity of CREB/ATF1soasto mimicking melanocyte-stimulating hormone signalling to induce expression of MITF [13] . In this kind of tumour MITF appears to have an oncogenic role as well [13] . Post-translational modification is important in regulation of MITF activity. As reviewed in ref. 1 , MITF is subject to multiple modifications. One is phosphorylation by MAPK [14] , which may occur as a consequence of receptor tyrosine kinase activity or other upstream signals in the RAS–RAF–MEK–ERK signalling cascade, resulting in MITF phosphorylation on serine 73. One important consequence of this phosphorylation is ubiquitin-dependent proteolysis of MITF [15] thereby linking MITF stability to MAPK pathway activity. Because activating mutational events within the MAPK pathway are particularly common in melanoma, it is plausible that MITF phosphorylation and ubiquitination are also common. Despite existing information about MITF's importance as a viability factor and its regulation by phosphorylation/ubiquitiation/degradation, little is known about the enzymes that catalyse MITF ubiquitination/deubiquitination reactions. In this study, we utilized a shRNA library against the known deubiquitinating enzymes (DUBs) to identify DUBs that deubiquitinate ubiquitin-MITF (ubMITF). The screen identified ubiquitin-specific protease 13 (USP13, also named Isopeptidase T-3) that upregulates MITF protein levels through stabilizing MITF protein via deubiquitination. Additionally, the stabilization of MITF by USP13 was found to be required for proliferation of melanoma cells and growth in soft agar, highlighting the importance of ubiquitin-mediated regulation of MITF activity in melanoma. Identification of USP13 To identify genes that are required for MITF deubiquintination, we utilized a shRNA library against DUBs to inhibit endogenous DUB expression. If a DUB was responsible for MITF deubiquitination, knockdown of the enzyme should enhance MITF degradation through favouring the ubiquitinated form, which is subject to proteosome-mediated degradation. shRNA constructs against 55 DUBs [16] and an expression vector encoding HA-tagged MITF were co-transfected into 293T cells and MITF protein levels were assessed 48 h later. A decrease in MITF protein level compared with shLuciferase (control) was seen with several shDUBs, with D1 being most dramatic ( Supplementary Fig. S1 ) as well as the most reproducible (data not shown). DUB D1 was confirmed by sequencing to be USP13 (ubiquitin-specific protease 13, also called ubiquitin-specific peptidase, isopeptidase T-3). To test whether shUSP13 reduces endogenous MITF protein levels, three hairpin shRNAs against USP13 were introduced into several human melanoma cell lines. 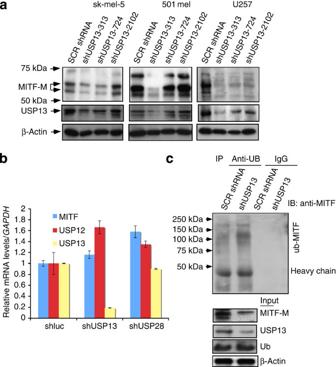Figure 1: Knockdown of USP13 post-transcriptionally reduces MITF protein levels and enhances ubiquitination of MITF in melanoma cells. (a) Melanoma cell lines sk-mel-5, 501mel and UACC257 (U257) were infected with lentivirus expressing shUSP13 (3 different targeting vectors named 313, 724, and 2102) or control shRNA (SCR shRNA). After 48 h of selection with G418, cells were collected for detection of MITF by western blot. A decrease in MITF protein was observed on USP13 knockdown. (b) 501mel cells containing shUSP13, shUSP28 or control shRNA (shluc) were collected for RNA isolation. The relative mRNA levels of MITF, USP13 and USP12 were detected by real-time RT–PCR. GAPDH was used as an internal reference. Data and error bars (s.d.) represent experiments carried out in triplicate. (c) 501mel cells were infected with shUSP13 (313) or control shRNA (SCR shRNA). After cell lysis and treatment with MG132, immunoprecipitation was performed using an anti-ubiquitin antibody. ubMITF was detected using anti-MITF antibody. As shown in Figure 1a , knockdown of USP13 produced proportional suppression of MITF protein levels. The clone shUSP13 (313) uses the same DNA sequence as the USP13-targeted DUB in the shRNA library. Similar effects on MITF levels were observed upon knockdown of USP13 in several extra melanoma cell lines ( Supplementary Fig. S2 ) Figure 1: Knockdown of USP13 post-transcriptionally reduces MITF protein levels and enhances ubiquitination of MITF in melanoma cells. ( a ) Melanoma cell lines sk-mel-5, 501mel and UACC257 (U257) were infected with lentivirus expressing shUSP13 (3 different targeting vectors named 313, 724, and 2102) or control shRNA (SCR shRNA). After 48 h of selection with G418, cells were collected for detection of MITF by western blot. A decrease in MITF protein was observed on USP13 knockdown. ( b ) 501mel cells containing shUSP13, shUSP28 or control shRNA (shluc) were collected for RNA isolation. The relative mRNA levels of MITF, USP13 and USP12 were detected by real-time RT–PCR. GAPDH was used as an internal reference. Data and error bars (s.d.) represent experiments carried out in triplicate. ( c ) 501mel cells were infected with shUSP13 (313) or control shRNA (SCR shRNA). After cell lysis and treatment with MG132, immunoprecipitation was performed using an anti-ubiquitin antibody. ubMITF was detected using anti-MITF antibody. Full size image To determine whether knockdown of USP13 influences the expression of MITF messenger RNA levels, 501mel cells were infected with shUSP13 (313), shUSP28 (specificity control) or scrambled control shRNA, followed by analysis of mRNA levels for MITF, USP13, and USP12 (specificity control) using quantitative RT–PCR. In contrast to the observed decrease in MITF protein levels upon USP13 knockdown, MITF mRNA levels were not decreased by these treatments, despite high efficiency of USP13 knockdown ( Fig. 1b ). This experiment suggests that USP13 regulates MITF expression posttranslationally. The expression of USP12 was not decreased by shUSP13 ( Fig. 1b ). To test the specificity of DUB enzymatic activity, shRNA against USP28 (ref. 17 ) was also employed but produced no significant effect on MITF expression ( Fig. 1b ). To test whether USP13 regulates MITF protein levels through regulation of its ubiquitination, extracts of 501mel cells containing shUSP13 (313) or scrambled shRNA were subjected to immunoprecipitation/western blotting. Once cells were lysed, the proteasome inhibitor MG132 was added to the cell lysate to prevent MITF from proteasome degradation in vitro . Immunoprecipitation was performed using an anti-ubiquitin antibody, followed by the detection of MITF (ubMITF) using C5 monoclonal antibody. As shown in Figure 1c , ubiquitinated MITF strongly accumulated in 501mel–shUSP13, suggesting that knockdown of USP13 inhibits deubiquitination of ubMITF. Taken together, these results are consistent with the possibility that USP13 has a significant role in modulating MITF levels through altering its state of ubiquitination. USP13 stabilizes and upregulates MITF We next examined whether USP13 influences MITF protein stability by introducing an expression vector for USP13 into U257 (UACC257) melanoma cells. Expression of HA-tagged cDNA encoding USP13 enhanced the steady-state levels of endogenous MITF ( Fig. 2a ). 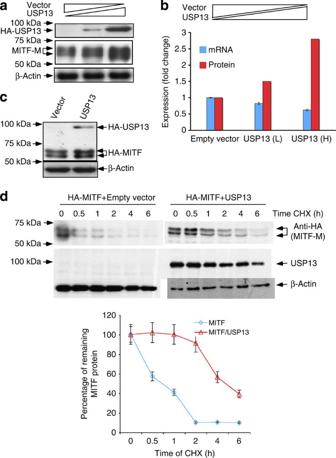Figure 2: Exogenous USP13 stabilizes endogenous and exogenous MITF. (a) U257 cells were transfected with HA-tagged USP13, followed by western blotting. Endogenous MITF protein levels increased in a dose-dependent manner. (b) U257 cells were transfected with USP13 as in (a). 24 h later, cells were collected for isolating RNA. The relative levels of MITF mRNA were detected by real-time RT–PCR. GAPDH was used for normalization. The MITF protein levels in panel (a) were measured and represented in same graph (β-actin was used for normalization). Exogenous USP13 increases MITF protein levels without increasing MITF mRNA levels. The label L: 100 ng USP13 plasmid per well; H: 500 ng USP13 plasmid per well in 6-well plate. (c) U257 cells were co-transfected with HA-tagged MITF and HA-tagged USP13, followed by western blotting using anti-HA antibody to detect both HA-tagged USP13 and HA-tagged MITF. USP13 increased exogenous MITF protein levels. (d) 293T cells were transfected with HA–MITF as well as either empty vector or USP13. The transfected cells were treated with cyclohexamide (CHX) and cells were collected at the indicated time points to measure levels of MITF protein. The MITF protein bands were quantified and normalized to β-actin. The apparent half-life of MITF was significantly extended on co-expression of USP13 (from 30 min to more than 4 h) consistent with an effect by USP13 on MITF protein stability. Quantification of HA–MITF protein levels (normalized to β-actin) is plotted in the accompanying graph. Error bars (s.d.) were calculated from three different measurements. As shown in Figure 2b , MITF protein levels increased significantly, whereas mRNA levels did not. To further assess the MITF-gene transcription-independence of USP13's effects, we co-transfected HA-tagged USP13 and MITF expression vectors into U257 cells. As shown in Figure 2c , USP13 overexpression was seen to upregulate protein levels of MITF driven off an exogenous promoter, further supporting a mechanism that is independent of MITF gene transcription. We next wished to assess the effect of USP13 on MITF protein stability. For this experiment, both HA-tagged MITF and USP13 were expressed in 293T cells by transient transfection. After 24 h, the synthesis of new proteins was blocked by cycloheximide, cells were collected at specific time points, and MITF protein levels were detected using anti-HA antibody. As shown in Figure 2d , the half-life of transfected MITF in the absence of USP13 was significantly shorter than in the presence of USP13. Quantification of the stability/kinetics is shown in Figure 2d . Figure 2: Exogenous USP13 stabilizes endogenous and exogenous MITF. ( a ) U257 cells were transfected with HA-tagged USP13, followed by western blotting. Endogenous MITF protein levels increased in a dose-dependent manner. ( b ) U257 cells were transfected with USP13 as in ( a ). 24 h later, cells were collected for isolating RNA. The relative levels of MITF mRNA were detected by real-time RT–PCR. GAPDH was used for normalization. The MITF protein levels in panel ( a ) were measured and represented in same graph (β-actin was used for normalization). Exogenous USP13 increases MITF protein levels without increasing MITF mRNA levels. The label L: 100 ng USP13 plasmid per well; H: 500 ng USP13 plasmid per well in 6-well plate. ( c ) U257 cells were co-transfected with HA-tagged MITF and HA-tagged USP13, followed by western blotting using anti-HA antibody to detect both HA-tagged USP13 and HA-tagged MITF. USP13 increased exogenous MITF protein levels. ( d ) 293T cells were transfected with HA–MITF as well as either empty vector or USP13. The transfected cells were treated with cyclohexamide (CHX) and cells were collected at the indicated time points to measure levels of MITF protein. The MITF protein bands were quantified and normalized to β-actin. The apparent half-life of MITF was significantly extended on co-expression of USP13 (from 30 min to more than 4 h) consistent with an effect by USP13 on MITF protein stability. Quantification of HA–MITF protein levels (normalized to β-actin) is plotted in the accompanying graph. Error bars (s.d.) were calculated from three different measurements. Full size image ubMITF is a substrate of USP13 Although our experiments suggest that USP13 stabilizes MITF and influences the level of ubMITF in cells, biochemical studies were carried out to more directly examine whether USP13 deubiquitinates MITF. Utilizing a 'TNT' in vitro coupled transcription/translation system, 35 S-labelled MITF and nonradioactive USP13 were produced in rabbit reticulocyte extracts (Promega). To make ubiquitinated MITF (ubMITF), polyubiquitin chain (UB 2–7 ; Boston Biochem) was conjugated to 35 S-MITF under the catalytic action of TIPP (Thermostable Inorganic Pyrophosphatase) and ATP [18] . To study the deubiquitinating activity of USP13, 35 S-ubMITF was mixed with USP13 to perform a deubiquitination assay [18] . Equal quantities of 35 S-MITF from each reaction were loaded onto SDS–PAGE gels for analysis. 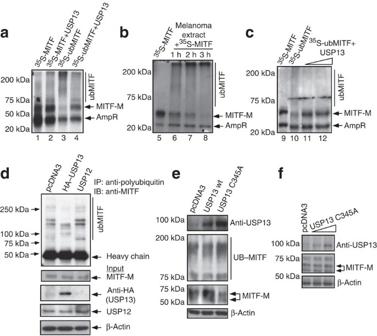Figure 3: Deubiquitination of MITF by USP13 is enzymatic-dependent. (a)In vitrotranscribed/translated35S-MITF (first lane) was ubiquitinated using TIPP (thermostable inorganic pyrophosphatase; third lane) and then incubated within vitrotranscribed/translated USP13 to perform deubiquitination reaction (fourth lane). An ampicillin-resistance protein band running below MITF is indicated by asterisk (is affected by the ubiquitination reaction, but not by USP13). (b)In vitrotranscribed/translated35S-MITF was incubated in a melanoma cell lysate containing ubiquitinating activity together with poly-ubiquitin chain and ubiquitin conjugating enzyme fractions. MITF levels decreased in a time-dependent manner while high molecular weight form(s) correspondingly appeared at the top of the gel, consistent with polyubiquitinated MITF. (c) Polyubiquitinated35S-MITF from (B, 1 h) was incubated with recombinant USP13. The high molecular weight (polyUb) MITF diminished and was associated with reappearance of free MITF. (d) U257 cells were transfected with pcDNA3, USP13 or USP12 and lysed after 3 days in the presence of MG132. Immunoprecipitation was performed by anti-poly-ubiquitin (FK2) antibody, followed by western blot detection using anti-MITF antibody to examinein vivodeubiquitination of MITF by USP13. Note that free MITF is not seen due to the ubiquitin-immunoprecipitation step. Diminished mobility forms are seen, consistent with deubiquitination of MITF in the presence of USP13. (e) U257 cells were transfected with wild-type USP13, USP13 C345A or empty vector and expressed for 3 days. Cells were treated with MG132 for 1 h before making lysates in the presence of MG132, followed by western blot using anti-USP13, anti-MITF and anti-β-ACTIN antibodies. (f) U257 cells were transfected with different doses of USP13 C345A or empty vector. After 3 days expression, cells were lysed in presence of MG132, followed by western blot using anti-USP13, anti-MITF and anti-β-actin. The results in Figure 3A demonstrate a high efficiency of MITF polyubiquitination (compare lanes 1 and 3) under the applied reaction conditions. ubMITF was seen to be efficiently deubiquitinated by USP13 (compare lanes 3 and 4) without influencing the nonubiquitinated 35 S-MITF pattern (compare lanes 1 and 2), suggesting that USP13 triggers MITF deubiquitination. Figure 3: Deubiquitination of MITF by USP13 is enzymatic-dependent. ( a ) In vitro transcribed/translated 35 S-MITF (first lane) was ubiquitinated using TIPP (thermostable inorganic pyrophosphatase; third lane) and then incubated with in vitro transcribed/translated USP13 to perform deubiquitination reaction (fourth lane). An ampicillin-resistance protein band running below MITF is indicated by asterisk (is affected by the ubiquitination reaction, but not by USP13). ( b ) In vitro transcribed/translated 35 S-MITF was incubated in a melanoma cell lysate containing ubiquitinating activity together with poly-ubiquitin chain and ubiquitin conjugating enzyme fractions. MITF levels decreased in a time-dependent manner while high molecular weight form(s) correspondingly appeared at the top of the gel, consistent with polyubiquitinated MITF. ( c ) Polyubiquitinated 35 S-MITF from (B, 1 h) was incubated with recombinant USP13. The high molecular weight (polyUb) MITF diminished and was associated with reappearance of free MITF. ( d ) U257 cells were transfected with pcDNA3, USP13 or USP12 and lysed after 3 days in the presence of MG132. Immunoprecipitation was performed by anti-poly-ubiquitin (FK2) antibody, followed by western blot detection using anti-MITF antibody to examine in vivo deubiquitination of MITF by USP13. Note that free MITF is not seen due to the ubiquitin-immunoprecipitation step. Diminished mobility forms are seen, consistent with deubiquitination of MITF in the presence of USP13. ( e ) U257 cells were transfected with wild-type USP13, USP13 C345A or empty vector and expressed for 3 days. Cells were treated with MG132 for 1 h before making lysates in the presence of MG132, followed by western blot using anti-USP13, anti-MITF and anti-β-ACTIN antibodies. ( f ) U257 cells were transfected with different doses of USP13 C345A or empty vector. After 3 days expression, cells were lysed in presence of MG132, followed by western blot using anti-USP13, anti-MITF and anti-β-actin. Full size image Because TIPP-catalysed ubiquitination of MITF is nonspecific, we set out to carry out the same deubiquitination assay utilizing a more native ubiquitination reaction to synthesize ubMITF. Since the E3 ligase involved in MITF ubiquitination is uncertain, we set up an experimental protocol in which melanoma cell lysate (to provide essential factors for MITF ubiquitination) was mixed with ATP, ubiquitin conjugating enzyme fractions (Boston Biochem) and 35 S-MITF. As the incubation proceeded, the amount of free 35 S-MITF decreased while the amount of ubMITF increased ( Fig. 3b , lanes 6–8). We utilized this method in all subsequent ubiquitination/deubiquitination experiments to produce ubMITF. Recombinant GST–USP13 protein was expressed and purified (Promega) for testing its deubiquitinating activity. Similar to the above results, ubMITF was largely deubiquitinated to free MITF on addition of recombinant USP13 ( Fig. 3c , lanes 10–12), demonstrating that ubMITF is a substrate of USP13 in vitro . To further investigate whether USP13-mediated deubiquitination of MITF is specific and occurs in melanoma cells, U257 cells were transfected with an expression vector for USP13, USP12 (as negative control), or empty vector. An expression vector for ubiquitin (driven by the CMV promoter) was co-transfected to provide enough ubiquitin to enhance detection of MITF ubiquitination. 72 h after transfection, cells were collected to make cell lysates for immunoprecipitation with anti-polyubiquitin (FK2) antibody beads (MBL), followed by detection of ubMITF by western blot utilizing anti-MITF monoclonal antibody (C5). As shown in Figure 3d, although only a small proportion of cellular MITF was ubiquitinated (minimal changes in non-ubiquitinated MITF), overexpression of USP13, but not USP12, significantly decreased the level of endogenous ubMITF, suggesting that USP13 promotes deubiquitination of ubMITF in vivo . As a specificity control, we wished to test the activity of a catalytically inactive mutant of USP13. To make such a mutant, we aligned USP13's amino-acid sequence to USP14, a DUB with a well-defined cysteine catalytic motif, and thereby identified cysteine 345 as the corresponding catalytically critical residue, mutating it to alanine (USP13 C345A). To test the enzymatic activity of this mutant, U257 cells were transfected with wild-type USP13, USP13 C345A or empty vector. After 3 days, cells were treated with MG132 for 1 h, followed by cell lysis and SDS–PAGE. As shown in Figure 3e, wild-type USP13 increased the levels of free MITF-M, whereas USP13 C345A did not (it actually decreased free MITF-M, and it may have a dominant negative activity). Transfection with different doses of USP13 C345A did not significantly influence MITF-M levels in U257 cells ( Fig. 3f ). These results suggest that USP13 regulates MITF protein levels through an enzymatically mediated mechanism. USP13 interacts with polyubiquitinated MITF To test whether endogenous USP13 and MITF interact in vivo , cell lysates from U257 cells with or without treatment by proteasome inhibitor (MG132, for 4 h) were subjected to immunoprecipitation/western blotting. We first attempted to use C5 antibody (anti-MITF monoclonal) for immunoprecipitation, combined with anti-USP13 antibody for blotting. However, although we were able to detect MITF in both the MG132-treated and untreated eluates, we were unable to detect USP13 in either eluate (data not shown). Our inability to detect USP13 might have been due to the relatively poor affinity of C5 monoclonal antibody to ubMITF. We then utilized the reciprocal approach, using anti-USP13 antibody to perform immunoprecipitation followed by western blot against MITF with the C5 antibody. Only polyubiquitinated MITF, but not the free form of MITF, was detected in IP eluates ( Fig. 4a ). In contrast M-MITF (non-ubiquitinated, running at ∼ 60–65kDa) was present in the IP-input lysate ( Fig. 4a ) indicating its lack of interaction with USP13. Inhibiting proteasome activity by MG132 increased the level of both ubMITF in the eluate and M-MITF in the unbound lysate. 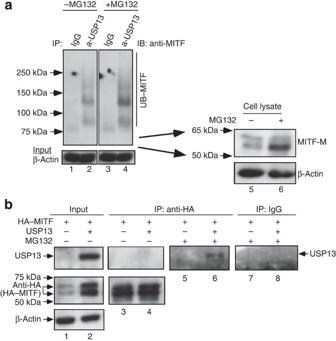Figure 4: USP13 interacts with ubMITF. (a) U257 cell lysates, with or without pretreatment with MG132, were immunoprecipated with anti-USP13 antibody, then detected using anti-MITF antibody. Only ubMITF interacts with USP13. (b) 293T cells were transfected with HA–MITF, USP13. Cells were collected and lysed. Immunoprecipation was done using anti-HA antibody, and detection of USP13 was done using anti-USP13 antibody. USP13 was only detected in the eluate from MG132 pretreated cell lysates. Figure 4: USP13 interacts with ubMITF. ( a ) U257 cell lysates, with or without pretreatment with MG132, were immunoprecipated with anti-USP13 antibody, then detected using anti-MITF antibody. Only ubMITF interacts with USP13. ( b ) 293T cells were transfected with HA–MITF, USP13. Cells were collected and lysed. Immunoprecipation was done using anti-HA antibody, and detection of USP13 was done using anti-USP13 antibody. USP13 was only detected in the eluate from MG132 pretreated cell lysates. Full size image To further attempt the reciprocal analysis, two expression vectors, one for HA-tagged MITF and one for USP13, were co-transfected into 293T cells. After 24 h of expression, cells were lysed for immunoprecipitation using anti-HA antibody, followed by detection of USP13 by western blot. Consistent with our previous results, USP13 was coimmunoprecipitated from the cell lysate with MG132 pretreatment (compare lanes 3, 4, 5 and 6 in Fig. 4b ) again suggesting that USP13 interacts selectively with ubMITF. Taken together, these results imply that only ubiquitinated MITF (ubMITF) interacts with USP13. USP13 regulates MITF target gene transcription We wished to test whether USP13 would influence MITF target gene expression. To this end, we isolated total RNA from 23 melanoma cell lines and 4 primary melanocyte lines from different donors, and performed real-time qRT–PCR to detect the mRNA levels of usp13 and Trpm1 (a known MITF target gene [19] ), using Glyceraldehyde-3-phosphate dehydrogenase ( GAPDH ) as internal reference. 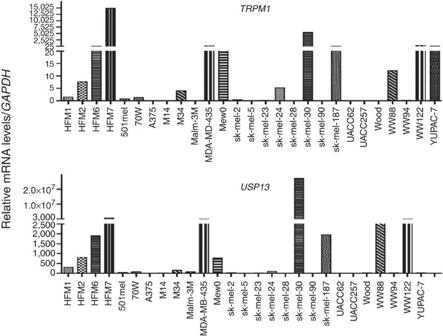Figure 5: Expression of USP13 and MITF targetTRPM1correlate in melanoma cell lines and in primary melanocytes. 23 melanoma cell lines and primary melanocytes from 4 donors were collected for RNA isolation. Real-time RT–PCR was applied for detecting the mRNA levels ofUSP13(bottom panel) andtrpm1(top panel).GAPDHwas used for normalization. The error bar was calculated from experiments carried out in triplicate. The correlation coefficientR=1.0 for malanocyte group,R=0.997 for melanoma cell group. As shown in Figure 5, expression levels of usp13 and Trpm1 correlated ( r =0.999 for melanocyte group, r =0.997 for melanoma cell group). To further determine whether USP13 activity would modulate MITF target gene expression, U257 melanoma cells were infected with two different shUSP13 vectors (constructs 313 and 724) or control shRNA, followed by measuring MITF target genes, Trpm1 and c-Met , mRNA by qRT–PCR. The levels of Trpm1 and c-Met mRNA were greatly reduced by knockdown of USP13 ( Fig. 6a ). In contrast, the levels of several non-MITF target genes, ( RARγ and Klf4 ) were not reduced. This relationship was further assessed by transfecting U257 melanoma cells with a Trpm1 promoter-driven luciferase reporter that was previously shown to be regulated by MITF [19] together with shUSP13 (313) or control shRNA. Twenty-four hours after transfection, cells were treated with DMSO or Forskolin, a cAMP agonist that upregulates expression of MITF and mimics the action of melanocyte stimulating hormone [7] . shUSP13 decreased both basal luciferase activity and the levels induced by Forskolin ( Fig. 6b ). Next, we assessed the effect of shUSP13 on MITF binding to the E-box in the endogenous Trpm1 promoter using ChIP assay ( Fig. 6c ). We observed that knockdown of USP13 reduces MITF binding at the Trpm1 promoter, whereas overexpression of MITF restores the diminished occupancy induced by shUSP13. Figure 5: Expression of USP13 and MITF target TRPM1 correlate in melanoma cell lines and in primary melanocytes. 23 melanoma cell lines and primary melanocytes from 4 donors were collected for RNA isolation. Real-time RT–PCR was applied for detecting the mRNA levels of USP13 (bottom panel) and trpm1 (top panel). GAPDH was used for normalization. The error bar was calculated from experiments carried out in triplicate. The correlation coefficient R =1.0 for malanocyte group, R =0.997 for melanoma cell group. 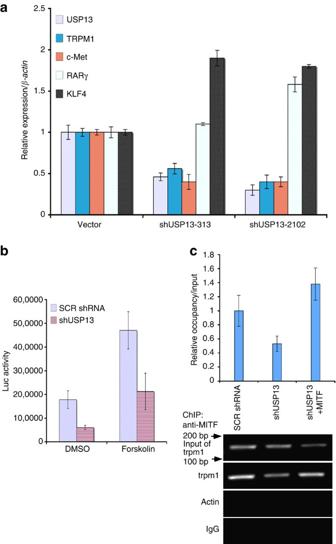Figure 6: USP13 regulates MITF target genes by influencing MITF binding to its target promoters. (a) RNA was isolated from U257 melanoma cells that were infected with lentiviruses targeting USP13. The expression of the MITF target genes,trpm1andc-met, as well as non-MITF target genes,RARγandKLF4, were detected by real-time RT–PCR. The error bars (s.d.) represent experiments carried out in triplicate. (b) U257 cells were transfected with TRPM1 promoter-driven luciferase reporters together with control shRNA or shUSP13(313). Cells were treated with DMSO or Forskolin in triplicate for 24 h before collecting for luciferase assay. Error bars indicate standard deviation (s.d.). Knockdown of USP13 decreases both basal and Forskolin-induced luciferase activity. (c) U257 cells containing control shRNA or shUSP13(313) were used for ChIP. After IP with anti-MITF antibody or IgG, the amount of trpm1 and actin promoter in the eluate was detected using semi-quantitative PCR (lower panels) and real-time PCR (upper panel). The error bar (s.d.) was calculated from triplicate data. Knockdown of USP13 reduced the binding of MITF to the trpm1 promoter. Full size image Figure 6: USP13 regulates MITF target genes by influencing MITF binding to its target promoters. ( a ) RNA was isolated from U257 melanoma cells that were infected with lentiviruses targeting USP13. The expression of the MITF target genes, trpm1 and c-met , as well as non-MITF target genes, RARγ and KLF4 , were detected by real-time RT–PCR. The error bars (s.d.) represent experiments carried out in triplicate. ( b ) U257 cells were transfected with TRPM1 promoter-driven luciferase reporters together with control shRNA or shUSP13(313). Cells were treated with DMSO or Forskolin in triplicate for 24 h before collecting for luciferase assay. Error bars indicate standard deviation (s.d.). Knockdown of USP13 decreases both basal and Forskolin-induced luciferase activity. ( c ) U257 cells containing control shRNA or shUSP13(313) were used for ChIP. After IP with anti-MITF antibody or IgG, the amount of trpm1 and actin promoter in the eluate was detected using semi-quantitative PCR (lower panels) and real-time PCR (upper panel). The error bar (s.d.) was calculated from triplicate data. Knockdown of USP13 reduced the binding of MITF to the trpm1 promoter. Full size image USP13 is required for cell proliferation and colony formation To determine whether USP13 activity influences growth/proliferation of human melanoma cells, U257 cells were infected with shUSP13 (313) or control shRNA. Cells were expanded with selection in a growth assay. After 5 days, U257 cells containing control shRNA were confluent. However, U257 cells containing shUSP13 (313) remained at significantly lower density ( Fig. 7a ), which represented ∼ 80% growth suppression. 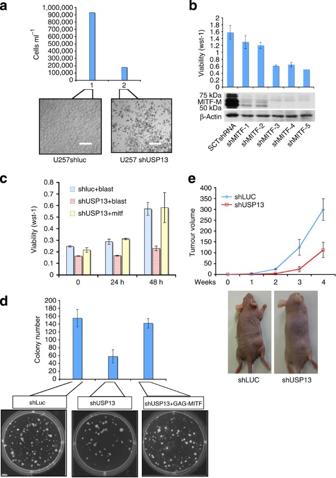Figure 7: Knockdown USP13 inhibits melanoma cell proliferation and colony formation. (a) U257SCR shRNA and U257shUSP13(313) were plated on 60 mm dishes with the density of 1×105cells and incubated at 37 °C for 5 days. USP13-depleted U257 cell growth was suppressed approximately 80%. Scale bar: 50 μm. (b) U257 cells were transfected with either of 5 different shMITF constructs or control shRNA in triplicate. Error bars indicate Standard deviation (s.d.). MITF knockdown resulted in decreased WST-1 signal. (c) Proliferation of U257shUSP13(313) cells was inhibited as measured by the WST1 assay. However, MITF overexpression in USP13-depleted U257 cells significantly rescues this proliferation inhibition. The data and error bars (s.d.) represent experiments carried out in triplicate. (d) U257shUSP13(313) and U257scr shRNA cells were suspended in soft-agar in triplicate and incubated at 37 °C for 3 weeks. The error bars represent standard deviation (s.d.). Colony formation for U257shUSP13 was 63% lower than for control cells (155±22 colonies in control wells compared with 58±17 colonies in the wells with shUSP13 cells. The studentt-test:P<0.0008). Introduction of MITF in USP13-depleted U257 cells rescued colony formation (up to 142±12 colonies). (e) Cells in D were injected subcutaneously into NCr nude mice. Xenograft tumour volume was measured once a week. Data points represent the mean±s.d. of 5 mice per group. Student'st-testPvalue=0.034. Representative xenograft tumours are shown. Figure 7: Knockdown USP13 inhibits melanoma cell proliferation and colony formation. ( a ) U257SCR shRNA and U257shUSP13(313) were plated on 60 mm dishes with the density of 1×10 5 cells and incubated at 37 °C for 5 days. USP13-depleted U257 cell growth was suppressed approximately 80%. Scale bar: 50 μm. ( b ) U257 cells were transfected with either of 5 different shMITF constructs or control shRNA in triplicate. Error bars indicate Standard deviation (s.d.). MITF knockdown resulted in decreased WST-1 signal. ( c ) Proliferation of U257shUSP13(313) cells was inhibited as measured by the WST1 assay. However, MITF overexpression in USP13-depleted U257 cells significantly rescues this proliferation inhibition. The data and error bars (s.d.) represent experiments carried out in triplicate. ( d ) U257shUSP13(313) and U257scr shRNA cells were suspended in soft-agar in triplicate and incubated at 37 °C for 3 weeks. The error bars represent standard deviation (s.d.). Colony formation for U257shUSP13 was 63% lower than for control cells (155±22 colonies in control wells compared with 58±17 colonies in the wells with shUSP13 cells. The student t -test: P <0.0008). Introduction of MITF in USP13-depleted U257 cells rescued colony formation (up to 142±12 colonies). ( e ) Cells in D were injected subcutaneously into NCr nude mice. Xenograft tumour volume was measured once a week. Data points represent the mean±s.d. of 5 mice per group. Student's t -test P value=0.034. Representative xenograft tumours are shown. Full size image MITF is known to have an important role in melanocyte survival and differentiation and is also an amplified oncogene in 10–20% of human melanomas [3] . Consistent with this finding, knockdown of MITF in U257 cells suppressed cell viability/metabolism as measured by WST-1 assay in a manner related to the level of MITF knockdown in each group ( Fig. 7b ). Similarly, knockdown of USP13 strongly inhibited U257 cell viability/metabolism ( Fig. 7c ), whereas introduction of MITF into the USP13-depleted U257 cells rescued cell proliferation. Similar proliferation and growth inhibition was observed in other melanoma cell lines (501mel cells, MALME-3M and SK-mel-5, data not shown). Taken together, these results are consistent with the model that USP13 can control melanoma cell proliferation through modulation of MITF activity. Next, soft agar colony assays were performed after shUSP13 or shUSP13+MITF. As shown in Fig. 7d , shUSP13 significantly suppressed melanoma cell colony formation, and its effect was rescued by simultaneous overexpression of MITF. Finally, we used xenograft tumour models to characterize USP13 knockdown in vivo . U257 cells with or without USP13 depletion were introduced into NCr nude mice. Partial USP13 knockdown suppressed growth of the tumour xenografts more than 60% ( Fig. 7e ). Collectively, these results suggest that USP13 functionally participates in the proliferative/growth-promoting activity of MITF in melanoma cells. MITF is required for melanocyte development and differentiation as well as melanoma cell survival and proliferation. Recent findings indicate that MITF is an oncogene and also has a role in melanoma development [3] . The biological functions of MITF in melanoma cells are likely to be determined at least in part by alterations in its protein level: high MITF protein levels are anti-proliferative and suppress melanoma cell invasion; medium levels are pro-proliferative; and low levels are required for melanoma-cell invasion [20] . In this study, we have identified the deubiquitination of MITF as a potent mechanism that regulates MITF protein turnover. The consequences of interfering with MITF deubiquitination appear to potently affect MITF target gene expression as well as growth/survival properties of melanoma cells, suggesting that this mechanism of MITF protein regulation is functionally important, at least in the setting of the melanoma cells studied here. Although MITF expression is transcriptionally regulated by multiple signalling pathways involved in melanoma development [1] , [21] , the ubiquitination and proteasome-mediated degradation of MITF suggests that ubiquitination/deubiquitination may also participate in regulating MITF function [15] . There is currently a shortage of data regarding enzymes responsible for MITF ubiquitination and deubiquitination. HUBC9 was initially suggested to be the E3 ligase responsible for MITF ubiquitination [18] . However, based on subsequent evidence that MITF is subject to SUMO modification, an activity strongly associated with HUBC9, it is more likely involved in that modification [19] , [22] . Further studies on the precise amino-acid targets of ubiquitination will also permit further mutational analyses to test stability influences on MITF activity. Here we identify USP13 as responsible for the deubiquitination of MITF. It has been found that protein ubiquitination has an important role in a number of biological processes such as cell development, differentiation, oncogenesis, cell cycle progression and transcriptional activation [23] , [24] , [25] , by regulating protein degradation. Our results show that the deubiquitination of MITF not only stabilizes and upregulates the activity of MITF, but also regulates MITF downstream target gene expression and increases melanoma cell proliferation and tumourigenesis. These findings highlight the important biological function of DUBs such as USP13. Before our work, USP13 was described as a functional yet uncharacterized DUB [26] . Based on structure analysis, USP13 belongs to a C-terminal 19 family of peptidases, containing 2 UBA (Ubiquitin-associated/translation elongation factor EF1B, amino-terminal) domains and one UBP (ubiquitin-specific processing protease)-type zinc finger domain. These structural features predict that USP13 can bind to ubiquitin and remove ubiquitin from its chain at the C-terminus. Recent evidence using mammalian systems as models have showed that some DUBs are important in the regulation of specific processes within mammalian cells. For instance, USP28 stabilizes cyclin E1 and c-Myc by counteracting the ubiquitination activity of SCF–Fbx7 ligase [17] . USP28 also has an important role in the control of DNA-damage-induced apoptosis via stabilization of Chk2 and 53BP1in response to DNA damage [27] , [28] . Another DUB named CYLD controls the NF-κB pathway by removing K63-linked polyubiquitin chains from several mediators of the cytokine-induced NF-κB pathway [29] , [30] . CYLD, as a tumour suppressor gene, is mutated in skin tumours (cylindromatosis), and was also found to be reduced or lack expression in human skin cancers as well as several other tumour types, including those of kidney, liver and uterine cervix, suggesting that CYLD may play a general role as a tumour suppressor. Our results indicate that the downregulation of USP13 by RNAi decreases both basal and Forskolin-mediated expression of MITF protein. The inhibition of MITF by shUSP13 appears to occur via the reduction of MITF deubiquitination and subsequent increase in MITF proteasome-mediated degradation. Melanoma cell proliferation was well correlated with endogenous MITF protein levels in shUSP13-treated cells. Furthermore, shUSP13-induced inhibition of cell proliferation and colony formation in soft-agar was rescued by exogenously expressed MITF. This result is in agreement with previously published work on MITF depletion in 501mel melanoma cells [3] . Taken together, these results indicate that USP13 has an important role in melanoma cells via regulation of ubiquitinated MITF. Further study of the expression and regulation of USP13 will improve our understanding of the physiological functions of USP13. In addition, correlative studies comparing MITF and USP13 protein levels will be important for further study and may help to determine if the influence of USP13 suppression would pertain to all melanomas rather than subsets of melanomas. In its role as a nuclear transcriptional factor, MITF is involved in multiple processes via its regulation of different transcriptional target genes [19] , [31] , [32] . The expression of the MITF target gene TRPM1 (ref. 19 ) is correlated with melanocytic tumour progression, melanoma tumour thickness, and the potential for melanoma metastasis [33] , [34] . Our results indicate that the expression of TRPM1 and USP13 are correlated in both melanocytes and melanoma cells. Additionally, we show that TRPM1 expression is regulated by USP13 through the modulation of MITF occupancy at the TRPM1 promoter. These results suggest a biological relationship between USP13 and MITF downstream target gene expression. Suppression of MITF activity could be therapeutically attractive in several settings: as a tissue-specific viability factor in melanoma, and as a central mediator of melanin production in settings of hyperpigmentation. However, MITF itself is a difficult drug target by standard criteria of 'drugability.' Enhancing MITF turnover by suppressing its deubiquitination potentially offers a promising approach. Our data suggest that USP13 slows turnover of MITF protein through deubiquitination, and thus regulates melanoma cell proliferation and tumourigenesis. On the basis of these results, the USP13 protease might be considered as a potential target for melanoma therapy. Cell culture and treatment Melanoma cell lines 501mel, U257 and SKMEL-5 were grown as described in McGill et al . [31] 293T cells were grown in Dulbecco's modified Eagle's medium supplemented with 10% fetal bovine serum and penicillin/streptomycin/ L -glutamine. For lentivirus infection, virus was produced in 293T cells according to the protocol described on the website of the Broad Institute ( http://www.broad.mit.edu ). The oligonucleotides of shUSP13 were cloned into pRNAtin6.1 (GenScript), and transfected into 293T cells using LipofectAMINE and Plus reagent (Invitrogen) as described in ref. 35 . Forty-eight hours after transfection, viruses were collected and used for infection of melanoma cells. After 3 days of selection, cells were collected for preparation of cell lysate or isolation of RNA. Transient and stable transfections were performed as described in Zhao et al . [35] For transient transfection, one-tenth amount of GFP vector was co-transfected to monitor and estimate the transfection efficiency under fluorescent microscopy. After transfection, cells were incubated for 3 days under the selection condition of 800 μg ml −1 G418 before collecting cells. For proliferation assays, WST-1 reagent was used according to the manufacturer's instructions (Roche). Plasmids For shRNA screening, the library that was cloned into pSUPER was provided by Dr. Rene Bernards (The Netherlands Cancer Institute), with each DUB targeted by four hairpins. The shRNA vectors for USP28 were purchased from Addgene; USP13, USP12 were purchased from Open Biosystems. To make the constructs against USP13, the blow sequences are targeted: shUSP13-313: AAGGGAACATGTTGAAAGACAT, shUSP13-724: GTGTGCCAGATGCGACCTGT, shUSP13-2102: GCATGTCGCAAGGCTGTGT. Immunoblotting Immunoblotting was performed as described in Wu et al . [15] After treatment as designed in each experiment, cells were lysed in lysis buffer containing MG132 (30 μM), followed by sonication at 20% power for 20 s. 8% SDS–PAGE gels were employed. The anti-USP13 (carboxy-terminal) was purchased from Abgent; the anti-β-actin was purchased from Santa Cruz; the anti-MITF monoclonal C5 antibody was produced within our laboratory. For quantification, the density of MITF bands were measured with AlphaImager 2200 (Alpha Innotech) and normalized to that of β-actin. Immunoprecipitation and chromatin immunoprecipitation assay Immunoprecipitation and chromatin Immunoprecipitation (ChIP) assays followed the procedures in Zhao et al . [35] For the ChIP assay, melanoma cells stably expressing shluc or shUSP13 (313) were cross-linked with 1% formaldehyde. Cell pellets were lysed and sonicated, and supernatants were diluted in IP buffer. After preclearing with 20 μg sheared salmon sperm DNA, 15 μl mouse IgG and 50 μl of 50% Protein A/G-agarose beads (Santa Cruz) were added, and immunoprecipitation was performed overnight at 4 °C with 20 μl of IgG or anti-MITF antibody. Complexes were recovered by 2 h incubation at 4 °C with 5 μg sheared salmon sperm DNA and 50 μl Protein A/G-agarose beads. Precipitation of chromatin complexes, reversal of formaldehyde cross-linking and purification of DNA fragments was done as described. 5 μl from a 50 μl DNA extraction was used per PCR reaction. The primers for amplifying TRPM1 promoter have been previously described [19] . For immunoprecipitation assay, cells were lysed in buffer containing 20 mM Tris at pH8.0, 1% Triton X-100, 250 mM NaCl and protease inhibitor cocktail. In vitro translation and ubiquitination/deubiquitination assays For in vitro translation of MITF and USP13, TNT T7-coupled rabbit reticulocyte lysate (Promega) was used under conditions recommended by the supplier. For covalent conjugate formation between MITF and Ub, the assay was performed as described in ref. 19 . For in vitro deubiquitination (deUB), 35 S-ubMITF was mixed with USP13 in deUB buffer (500 mM Tris–HCl. pH8.3, 250 mM KCl, 50 mM MgCl, 10 mM DTT), incubated at 37 °C for 1 h. The products were loaded on SDS–PAGE gels for separation, followed by fixing, enhancing and autoradiography. For cell lysate based in vitro deUB assays, the ubiquitinating reaction was processed in 20 μl containing 1 μl 100 mM creatine, 1 μg μl −1 creatine kinase, 100mM ATP, ubiquitin conjugating enzyme fractions (Sigma), 6 μl melanoma cell lysate, 2 μl 35 S-MITF and 3 μl ubiquitin chain (Boston Biochem) in the presence of MG132 (30 μM). The rest of the procedure is the same as above. Real-time quantitative RT–PCR Total RNA was isolated from cells with or without treatment according to the experimental design using Trizol reagent (Invitrogen). 100 ng total RNA was used in each reaction. The total volume for each reaction was 20 μl, including 10 μl ×2 Quanti PCR Master Mix (Bio-Rad), 0.12 μl QuantiTect RT Mix (Qiagen), and 0.5 μl of each primer (10 μM stock) with triplicates for each sample. Reverse transcription proceeded at 48 °C for 30 min, followed by 10 min at 95 °C to activate DNA polymerase. Forty cycles of PCR were then carried out at 95 °C for 15 s and 60 °C for 30 s. Real-time PCR was carried out using 7700 Fast (Applied Biosystem). The primers for USP13 were qUSP13-F: 5′-GGTCTACAAGAACGAGTG-3', QUSP13-R: 5′-TTCTCTCGCGCATGTCTT-3′. The primers for MITF, TRPM1, GAPDH were previously described in Miller et al ., 2004 (ref. 19 ) and McGill et al ., 2006 (ref. 31 ). Soft agar assay Cells (1,000 cells per well) were seeded in 0.32% low-melting point agarose (Sigma) in DMEM with 10% FBS, layered onto 0.64% agarose in DMEM with 10% FBS in 6-well plates. After cooling, 0.5 ml DMEM growth medium was added to the gel layer and incubated at 37 °C for 3 weeks. Colonies were stained with crystal violet, counted and photographed using a gel-Imager system. Xenograft tumour models Animal experiments were carried out according to IRB approved protocol that is in compliance with MGH and NIH guidelines. The human U257 melanoma tumour cells expressing control shRNA and shUSP13 were trypsinized and suspended in RPMI1640 growth medium. 1×10 6 cells in 50 μl were injected subcutaneously into the rear back of an NCr nude mouse. Five mice were injected per group. Tumour volume was measured once a week. Statistical significance was determined with a 2-tail Student's t -test. How to cite this article: Zhao, X. et al . Regulation of microphthalmia-associated transcription factor stability by the USP13 deubiquitinase. Nat. Commun. 2:414 doi: 10.1038/ncomms1421 (2011).